Mechano-actuated ultrafast full-colour switching in layered photonic hydrogels Photonic crystals with tunability in the visible region are of great interest for controlling light diffraction. Mechanochromic photonic materials are periodically structured soft materials designed with a photonic stop-band that can be tuned by mechanical forces to reflect specific colours. Soft photonic materials with broad colour tunability and fast colour switching are invaluable for application. Here we report a novel mechano-actuated, soft photonic hydrogel that has an ultrafast-response time, full-colour tunable range, high spatial resolution and can be actuated by a very small compressive stress. In addition, the material has excellent mechanical stability and the colour can be reversibly switched at high frequency more than 10,000 times without degradation. This material can be used in optical devices, such as full-colour display and sensors to visualize the time evolution of complicated stress/strain fields, for example, generated during the motion of biological cells. Photonic crystals are materials made from nanoscale periodic structures that cause Bragg diffraction to light of specific wavelength, producing colour. As photonic crystals constructed from soft materials, such as rubbers and gels, have the potential to change their periodicity through electrical [1] , [2] , magnetic [3] , chemical [4] , [5] , thermal [6] or mechanical stimuli [7] , [8] , [9] , they are drawing great attention for use as sensors [10] , [11] , [12] , [13] . For many applications, such as movie displays or fast responsive sensors, both full-colour tunability and video-rate fast colour switching are invaluable [9] , [14] . Many photonic gel materials, with a relatively broad range of colour tunability have been developed [5] , [11] , [12] . However, the reported response time of these materials, ranging from several seconds to a few hours, is much slower than the video rate [12] , [14] , [15] , [16] . The colour tuning of the gel materials can be classified into two mechanisms. One is based on the volume change due to swelling/deswelling of gel materials upon various external stimuli. Governed by solvent diffusion, the response time in this case increases with the sample size squared, and thus it becomes very slow for bulk samples [17] . The other is based on the mechanical deformation. The existing mechanochromic photonic materials usually have slow colour switching ability due to their strong time-dependent mechanical behaviour [13] , [18] . So the strategy to develop fast colour switching photonic materials is to use elastic soft materials that can deform and recover instantly in response to stress on and off without any delay. The time-dependent mechanical behaviour of a gel comes from viscoelasticity and poroelasticity [19] , [20] . The rearrangement of polymer chains and reversible crosslinks contribute to viscoelasticity and the relaxation time ( τ v ) is related to the shear viscosity ( η ) and the shear modulus of the gel ( μ ) by [19] , τ v = η / μ . Gels containing dynamic physical bonds, including most of existing photonic gels, have long relaxation times due to their high shear viscosity. In contrast, for chemically crosslinked gels that are highly swollen in good solvents, there are no appreciable physical bonds in the gels. So the longest relaxation time is from the Rouse mode relaxation of the crosslinked polymer chains [19] . In this case, the shear viscosity, η , is close to that of the solvent, and the viscoelastic relaxation time is extremely short. For example, considering a chemical hydrogel with μ =1 kPa, η= 10 −3 Pa s (water), the viscoelastic relaxation time τ v =10 −6 s. So chemically crosslinked gels may have fast mechanical response. The poroelasticity is associated with the solvent flow in gels and its relaxation time ( τ p ) is related to the characteristic size of the gel ( d ) and collective diffusion coefficient of the polymer network ( D c ) by Suzuki et al . [21] , τ p = d 2 / π 2 D c . For example, a typical polyacrylamide gel with a thickness d =1 mm, and D c ≃ 10 −10 m 2 s −1 , has a poroelastic relaxation time τ p =10 3 s. Thus, for a bulk chemical gel, τ p ≫ τ v . When the deformation rate (compression velocity/sample thickness) is fast enough such that , the poroelasticity is negligible and the gel can be treated as incompressible. On the other hand, when is low enough such that , the viscoelasticity is negligible and gel exhibits quasi-elastic behaviour. That is, a bulk chemical hydrogel will exhibit quasi-elastic behaviour and show instant mechanical response in the deformation rate of . As the τ v of a chemical gel is so short, the gel can maintain the elastic behaviour even at a very high deformation rate. Thereby, high water content chemical hydrogels have a great potential as mechanochromic materials possessing fast along with a broad colour switching ability. Then, the challenge is how to incorporate the photonic structure while maintaining the quasi-elastic nature of the hydrogel in the designed deformation rate. In this paper, we present a bio-inspired strategy to design the structure of quasi-elastic photonic materials from hydrogels. Based on this structure design, we developed a high water content, soft photonic hydrogel that has an ultrafast-response time (~0.1 ms) to mechanical compression. In addition, the gel also has a large reversible colour spectra range (340–640 nm), high spatial resolution (~10 μm), excellent mechanical stability (>10 4 cycling test) and can be actuated by very small compressive pressures (<3 kPa). We anticipate that these ultrafast colour tunable materials will find application in displays, highly sensitive stress sensor or telecommunication devices. Fabrication of photonic hydrogels with reflection platelets Inspired from the structure of colourful tropical fishes, we present a strategy to design the fast responsive photonic hydrogels. Many tropical fishes show bright structural colour that can undergo dramatic and lightning-quick transformations in response to environmental stimuli. In these fish scales, many rigid platelets of ~10 μm are periodically embedded in soft matrix to reflect light, and the quick colour change is caused by the spacing or angle variation between the reflective platelets [22] , [23] ( Fig. 1a ). So if one can embed ‘reflective platelets’ with periodically layered structure in a chemically crosslinked hydrogel matrix, the rigid platelets would selectively diffract light by interference; and the soft, elastic matrix would rapidly deform to change the interlayer spacing of platelets in response to the applied stress ( Fig. 1b ). 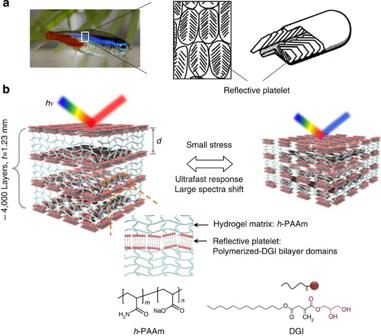Figure 1: Bio-inspired ultrafast colour tuning of the photonic hydrogel. (a) Image of a tropical fish neon tetra, and its photonic structure (reproduced from ref.22with permission). (b) Inspired bya, this work develops a photonic hydrogel, which contains alternative stacking of rigid polymerized-DGI bilayer domains in the soft, chemically crosslinked hydrogel from hydrolyzed (h)-PAAm. The rigid bilayer domains with inter-bilayer distance of 150–250 nm, acting as ‘reflective platelets’, selectively diffract visible light by interference, and the h-PAAm gel layers are quasi-elastic and deform rapidly in response to the applied stress. Thus, the nanostructured hydrogel exhibits a unique combination of ultrafast-response time, full-colour tunability, low actuating stress and excellent mechanical stability. Figure 1: Bio-inspired ultrafast colour tuning of the photonic hydrogel. ( a ) Image of a tropical fish neon tetra, and its photonic structure (reproduced from ref. 22 with permission). ( b ) Inspired by a , this work develops a photonic hydrogel, which contains alternative stacking of rigid polymerized-DGI bilayer domains in the soft, chemically crosslinked hydrogel from hydrolyzed ( h )-PAAm. The rigid bilayer domains with inter-bilayer distance of 150–250 nm, acting as ‘reflective platelets’, selectively diffract visible light by interference, and the h-PAAm gel layers are quasi-elastic and deform rapidly in response to the applied stress. Thus, the nanostructured hydrogel exhibits a unique combination of ultrafast-response time, full-colour tunability, low actuating stress and excellent mechanical stability. Full size image The ultrafast-response photonic hydrogels with platelets is developed based on a photonic hydrogel consisting of uniaxially aligned bilayers and chemically crosslinked hydrogel matrix named as PDGI/PAAm hydrogel. Here, PDGI stands for the homo-polymerized poly(dodecyl glyceryl itaconate) amphiphilic bilayers of ~5 nm thick and PAAm is polyacrylamide hydrogel layers of hundred nanometre thickness [11] . Since the bilayers are formed by hydrophobic association, they are strongly viscoelastic. As a result, the PDGI/PAAm hydrogel exhibits a relaxation time longer than 10 min under a loading–unloading deformation cycle [18] , which leads to very slow colour response ( Supplementary Fig. 1 ). The response of this gel can be improved by introducing an interpenetrating network structure of the PAAm hydrogel layers. However, it still took ~15 s for colour recovery [15] . Mimicking the platelet structure in tropical fishes, we need to split the rigid, continuous bilayers into small domains. By doing so, the bilayers do not deform during compression but only contribute to the reflection of light, which result in an ultrafast-response and broad wavelength tunable photonic hydrogel ( Supplementary Fig. 1 ). This was done by means of a post-modification hydrolysis reaction, which converts some amide groups in PAAm gel layers into carboxyl groups, providing sodium polyacrylate (See experimental section for detail, and Supplementary Fig. 2 ). The partially hydrolyzed PAAm gel layers, named as h-PAAm, carry charges and exert high ionic osmotic pressure to substantially swell the gel, particularly along the direction of layers. Such large anisotropic swelling splits the continuous bilayers into small domains. 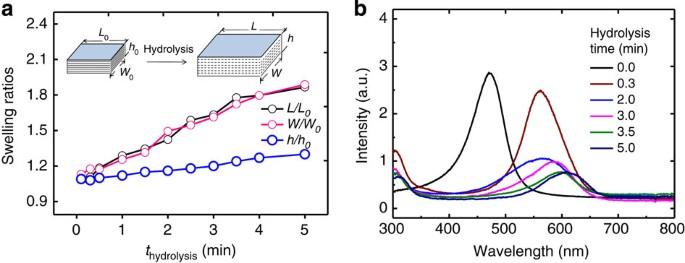Figure 2: Swelling behaviour and reflection spectra of the hydrogels with hydrolysis. (a) Different time of hydrolysis results in varying swelling ratios of the gel in two directions: along or normal to the layers. The swelling along the layers (W/W0,L/L0) is much larger than the swelling normal to the layers (h/h0). (b) Along with the swelling behaviour, the colour of the gel shows different levels of red shift, which can effectively be seen from the wavelength peak shift of the gel. All of the reflection spectra was measured at an incident angle of 60°. The sample thinckness before hydrolysish0was 0.97 mm. Figure 2a shows the anisotropic swelling behaviour of the gel treated with different hydrolysis time. For PDGI/PAAm sample before hydrolysis, the swelling along the layer direction has been completely constrained due to water impermeable nature of the bilayers. Gradual hydrolysis exerts high osmotic pressure to split the rigid, un-swellable PDGI layers into small domains and releases this swelling constraint. Thus, the swelling along the layer is much larger than that normal to the layers ( Fig. 2a ). By hydrolysis, the thickness of the sample increased from 0.97 mm ( t hydrolysis =0) to 1.23 mm ( t hydrolysis =5 min). Although breaking of the bilayers causes certain broadening of the spectrum ( Fig. 2b ), the hydrolyzed samples (PDGI/h-PAAm) still show a bright colour with a red shift due to the increase in the layer distance. The sharp angle dependence of the colour and the 2nd order diffraction peak shown in Supplementary Fig. 3 , indicate that the split bilayer domains serve as excellent platelets to diffract light. Figure 2: Swelling behaviour and reflection spectra of the hydrogels with hydrolysis. ( a ) Different time of hydrolysis results in varying swelling ratios of the gel in two directions: along or normal to the layers. The swelling along the layers ( W/W 0 , L/L 0 ) is much larger than the swelling normal to the layers ( h/h 0 ). ( b ) Along with the swelling behaviour, the colour of the gel shows different levels of red shift, which can effectively be seen from the wavelength peak shift of the gel. All of the reflection spectra was measured at an incident angle of 60°. The sample thinckness before hydrolysis h 0 was 0.97 mm. Full size image Large deformation and hysteresis behaviours These photonic hydrogels are free-standing and robust enough to allow mechanical compression. The original structural colour can be tuned by using proper amount of chemical cross-linker density of the hydrogel matrix. To induce a colour change across the whole visible range, from red ( λ max =640 nm) to blue ( λ max =340 nm), the maximum compressive strain required is estimated to be ε =Δ h / h =Δ λ max / λ max =0.5, where h , Δ h , Δ λ max are the thickness, change of thickness, and change of peak wavelength, respectively. The cyclic compressive test up to a strain ε =0.5 is performed at a loading/unloading velocity of 0.5 mm s −1 . The PDGI/PAAm gel shows an appreciable hysteresis ( Fig. 3a ), indicating energy dissipation due to the breakage of the non-covalent hydrophobic bonds of the bilayers upon deformation [18] . Though the broken hydrophobic bonds can reform, it takes a long time ( Supplementary Movie 1 ). As shown in Fig. 3d , the unloading curve could not recover to the intact initial state within the unloading time (1.2 s), and a residual strain remains at zero stress. As a result, during subsequent immediate compression, the stress–strain curves cannot completely superpose on the first cycle. It takes >6 min to recover to the original stress–strain curve after removal of the compressive strain ε =0.5 (corresponding to a stress of ~10 kPa). After hydrolysis, the PDGI/h-PAAm gel becomes soft and elastic, and the hysteresis area of the gel decreases gradually with the increase of hydrolysis time, indicating that less bilayers are broken during deformation ( Fig. 3b,c ). By hydrolysis, the stress–strain curves begin to overlap with the initial one ( Fig. 3e,f ). Especially when the hydrolysis time is 5 min, the stress–strain curves are completely superposed to the initial one, suggesting a full recovery of the hydrogel structure within the unloading time period of 1.2 s, although a small hysteresis is still observed ( Fig. 3c,f ). As we also observed some hysteresis for pure PAAm gel that is elastic, this small hysteresis partially comes from interface sliding friction between the gel and the machine during compression. The full recovery of the hysteresis within the unloading time suggests that the PDGI/h-PAAm hydrogel hydrolyzed for 5 min will exhibit complete recovery of deformation at a time scale significantly shorter than the unloading time of the tensile machine. 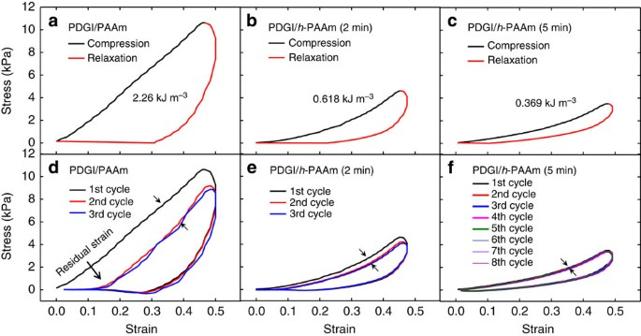Figure 3: Cyclic stress–strain curves of the photonic hydrogels. Samples with different hydrolysis time,thydrolysis(a–c: 0 min, 2 min, 5 min, respectively) show different cyclic stress–strain curves and hysteresis behaviours. The area of the hysteresis loop is the energy dissipated due to rupture of the hydrophobic association of the PDGI bilayers. The sample with long hydrolysis time (5 min) becomes soft and elastic, with a small hysteresis area (0.37 kJ m−3). Successive cyclic curves (d–f) are performed for several cycles. The hysteresis loops do not superpose for samples with little or no hydrolysis. While the sample with longer hydrolysis time (thydrolysis=5 min) shows completely superposed hysteresis loops even for more than eight cycles. Thus, the recovery time should be shorter than the unloading time of the tensile machine that is 1.23 mm × 0.5/0.5 mm s−1=1.2 s (thickness=1.23 mm, strain=0.5, loading/unloading velocity=0.5 mm s−1). Figure 3: Cyclic stress–strain curves of the photonic hydrogels. Samples with different hydrolysis time, t hydrolysis ( a – c : 0 min, 2 min, 5 min, respectively) show different cyclic stress–strain curves and hysteresis behaviours. The area of the hysteresis loop is the energy dissipated due to rupture of the hydrophobic association of the PDGI bilayers. The sample with long hydrolysis time (5 min) becomes soft and elastic, with a small hysteresis area (0.37 kJ m −3 ). Successive cyclic curves ( d – f ) are performed for several cycles. The hysteresis loops do not superpose for samples with little or no hydrolysis. While the sample with longer hydrolysis time ( t hydrolysis =5 min) shows completely superposed hysteresis loops even for more than eight cycles. Thus, the recovery time should be shorter than the unloading time of the tensile machine that is 1.23 mm × 0.5/0.5 mm s −1 =1.2 s (thickness=1.23 mm, strain=0.5, loading/unloading velocity=0.5 mm s −1 ). Full size image In the further study, we use the 5 min hydrolyzed sample, which has a water content of 95wt%, thickness 1.23 mm, Young’s modulus 3.2 kPa and shear modulus ~1 kPa. Ultrafast colour switching The fast colour switching properties of the PDGI/h-PAAm gel is first confirmed by the response of the hydrogel to step-wise compression-relaxations under a piece of glass driven manually. As shown in Supplementary Movie 2 , the red-coloured PDGI/h-PAAm gel shows instant full spectrum colour change in response to the compression and releasing. Furthermore, a gradient colour can be observed in response to a gradient stress field. As the manual compression is too slow to show the fast response of the gel, we design a ballistic test to observe the response of the gel when it is subjected to high velocity impacts. As shown in Fig. 4a , an air gun using 5-mm diameter plastic spheres as bullets is fired at a rubber film in front of the gel. The high-speed vibration of the rubber film is transmitted to the gel, and the deformation as well as colour change of the gel are recorded by a high-speed camera with a time resolution of 0.1 ms. The movie demonstrating the fast colour response to bullet fire is shown in Supplementary Movie 3 , which is replayed at 1/330 of the real speed. A vibration of the gel, with an elastic wave speed of ~m s −1 , was clearly observed. With the elastic wave regularly propagated from periphery to the centre, the gel changes colour from red to green with an unprecedented quick response. Images showing the behaviour of the gel over time are extracted from the high-speed footage ( Fig. 4b ). The colour of the gel changes between the neighbouring images with interval time about 0.3–0.6 ms, indicating that the colour switching rate reaches the order of ~0.1 ms. This colour switching rate should be related to the elastic wave velocity. The transverse wave velocity of the gel is a material parameter related to the shear modulus ( μ ) and the density of the gel ( ρ ) by Shearer [24] , c s =( μ / ρ ) 1/2 . For this gel, μ =1 kPa and ρ= 10 3 kg m −3 , c s =1 m s −1 , which is in consistent with the observation ( Supplementary Movie 3 ). The transverse wavelength, λ s , is sample geometry dependent. As the colour switching time is related as t ~ λ s / c s , the response rate can be further increased by decreasing the lateral sample size. On the other hand, the switching time by a mechanical indenter is related to the thickness of the sample ( h ), the compressive strain ( ε ), and the longitudinal wave velocity c l =(3 μ / ρ ) 1/2 , as t ~ εh / c l . For a sample of h =1 mm, the highest response rate to have full-colour switching ( ε =0.5) is c.a. 0.3 ms. Decreasing of the sample thickness will increase this response rate. 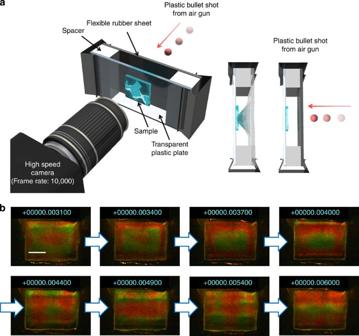Figure 4: Ultrafast colour tuning of the photonic hydrogel. (a) Schematic illustration of the ballistic impact test. The gel sample was placed in the centre of a transparent plastic plate. Five-millimetre diameter plastic spheres were used as bullets, and were fired against the rubber film by an air gun. The impact deformed the rubber and transmitted high-speed vibration to the sample, which cause the elastic waves of the gel accompanied with colour change. The fast elastic deformation and the colour change of the gel were captured by a high-speed camera (10,000 fps). (b) The images were extracted from the high-speed footage. The time elapsed was recorded on the top of the images automatically. The time interval between the neighbouring images was 0.3–0.6 ms. PDGI/h-PAAm hydrogel with hydrolysis time of 5 min was used, and the thickness of the hydrogel was 1.23 mm. Scale bar, 10 mm. Figure 4: Ultrafast colour tuning of the photonic hydrogel. ( a ) Schematic illustration of the ballistic impact test. The gel sample was placed in the centre of a transparent plastic plate. Five-millimetre diameter plastic spheres were used as bullets, and were fired against the rubber film by an air gun. The impact deformed the rubber and transmitted high-speed vibration to the sample, which cause the elastic waves of the gel accompanied with colour change. The fast elastic deformation and the colour change of the gel were captured by a high-speed camera (10,000 fps). ( b ) The images were extracted from the high-speed footage. The time elapsed was recorded on the top of the images automatically. The time interval between the neighbouring images was 0.3–0.6 ms. PDGI/h-PAAm hydrogel with hydrolysis time of 5 min was used, and the thickness of the hydrogel was 1.23 mm. Scale bar, 10 mm. Full size image As the original PDGI/PAAm gel has a response time of 10 min, the response rate is enhanced at least by a factor of 10 6 in the case of PDGI/h-PAAm gel. To the best of our knowledge, this is the fastest response reported so far for mechanochromatic photonic gels [7] , [12] , [15] , [25] , [26] . Full-wavelength colour tuning and high spatial resolution The respective reflection spectra at different compressive strains are shown in Fig. 5a . The reflection spectra shifted from red to blue with the increase in strain. Interestingly, the width of the spectra peak became narrow with the increase in the strain, indicating that the partially fluctuated bilayer domains become well-ordered again under an external stress. The peak wavelength of the spectra shows a linear dependence on the compressive strain ( ε ) over the whole visible spectrum range (640–340 nm) ( Fig. 5b ). 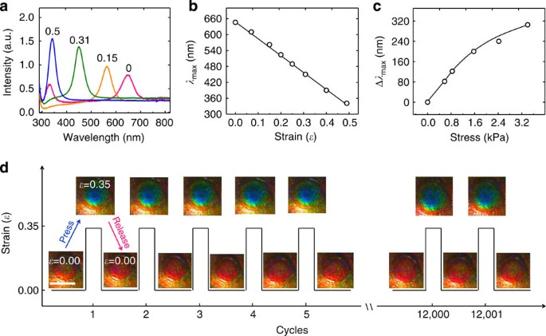Figure 5: Large colour tuning by small actuating stress and excellent mechanical stability. (a) The reflection spectra of the photonic gel under different compressive strain (ε). The peak wavelength,λmax, shows blue shift with an increase inε. (b) Theλmaxdecreases linearly with increasingε. (c) The relationship between the compressive stress and spectra wavelength shift, Δλmax. A compressive stress of 3.0 kPa (3 nN μm−2) can cause a blue shift of Δλmax=300 nm, from 640 to 340 nm. (d) The cycles of loading and unloading can be repeated for more than 12,000 times without degradation of the colour quality. The loading was driven by a rectangular oscillating system (frequency 100 Hz). Scale bar, 5 mm. Figure 5: Large colour tuning by small actuating stress and excellent mechanical stability. ( a ) The reflection spectra of the photonic gel under different compressive strain ( ε ). The peak wavelength, λ max , shows blue shift with an increase in ε . ( b ) The λ max decreases linearly with increasing ε . ( c ) The relationship between the compressive stress and spectra wavelength shift, Δ λ max . A compressive stress of 3.0 kPa (3 nN μm −2 ) can cause a blue shift of Δ λ max =300 nm, from 640 to 340 nm. ( d ) The cycles of loading and unloading can be repeated for more than 12,000 times without degradation of the colour quality. The loading was driven by a rectangular oscillating system (frequency 100 Hz). Scale bar, 5 mm. Full size image The rupture of the bilayers into small platelets by anisotropic swelling not only dramatically reduces the response time but also reduces the stiffness of the gels. The latter means a small stress is sufficient to deform the gel and cause colour change. As illustrated in Fig. 5c , the Δ λ max increases with the stress non-linearly due to the hyperelastic property of the hydrogel, and a compressive stress ( σ ) of 3.0 kPa can cause a blue shift of the peak wavelength Δ λ max =300 nm, across the full-colour range. This gives a stress sensibility (Δ λ max / σ ) as high as ~0.1 nm Pa −1 . To the authors’ knowledge, this is the most sensitive mechanochromatic photonic gel reported so far [9] , [13] , [26] , [27] , [28] . Ozin group has developed very attractive mechanochromatic elastic photonic crystals that can be used in fingerprinting, in which a stress of 15 kPa induced a blue shift of the peak wavelength ~80 nm (stress sensibility of 0.005 nm Pa −1 ) [7] . To demonstrate the high spatial resolution of the PDGI/h-PAAm gel, we place a human hair about 80 μm in diameter under a piece of glass and the red-coloured gel. When we manually moved the hair back and forth, a yellow line with a sharp boundary of the hair diameter appeared in the gel ( Supplementary Movie 4 ). This result indicates that the spatial resolution of the sample is within 80 μm. High fatigue resistance and repeatability The PDGI/h-PAAm gel has an excellent repeatability of colour switching, which is showed by a fatigue test using an experimental set up ( Supplementary Fig. 4 ). Supplementary Movies 5 and 6 show the colour change of the gel (at the first 20 cycles and last 20 cycles) in the fatigue test lasted for 12,000 loading–unloading cycles, and the corresponding static images are shown in Fig. 5d . The colour of the gel blue shifts upon loading and recovers by unloading. These results show that the mechanochromic switching behaviour can be repeated for more than 10,000 times without any noticeable changes in the optical properties. The amazing high fatigue resistance of this hydrogel, containing 95wt% of water, is related to the bilayer domains. Although the bilayer domains serve as rigid platelets at relatively small strain to reflect colour, they also serve as sacrificial bonds to dissipate energy at relatively large deformation, and thereby prevent the crack propagation and reinforce the soft gel [18] . Applications as pressure-actuated full-colour displays To demonstrate the potential application of this material as mechano-driven display, we further fabricated a simple display device as shown in Fig. 6a , which consists of the PDGI/h-PAAm gel and a glass plate embossed with the letters ‘LSW’. The dynamic behaviour of the gel in response to compression by the glass plate can be seen on video ( Supplementary Movie 7 ), and their static images are shown in Fig. 6b . Each individual frame is specific for a particular applied pressure. As shown in the pictures, the green-blue letters ‘LSW’ with sharp edges appear distinctly when the gel is pressed by the glass plate. As the gel is very sensitive to stress, a slight gradient in the stress distribution on the gel can induce gradient colour change. The intense gradient colour can appear not only in the ‘LSW’ region but also in the background. We can easily control the colour band tuning direction from top to bottom, left to right, or even in a diagonal direction depending on the direction of the stress distribution, which is unprocurable in common photonic materials, such as the PDGI/PAAm gel. The macroscopic patterns switched by subtle change in stress are remarkable and, to our knowledge, not have been found in other photonic materials. By using this hydrogel we can display, in principle, any picture. As shown in Fig. 6c , an oil painting-like picture including the sea, a boat and the sun vividly appears on the same gel by using an embossed glass plate with a pre-designed pattern. 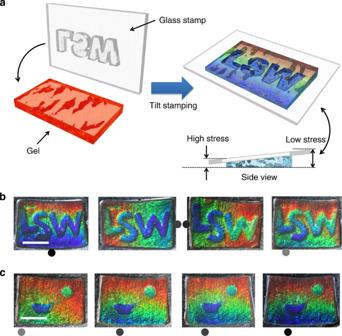Figure 6: A demonstration of the fast response photonic hydrogel as pressure-actuated full-colour displays. (a) A schematic illustration of pressure-actuated display. The elastic PDGI/h-PAAm gel (thydrolysis=5 min) was ~1.23 mm in thickness, and the pressure was given by a glass plate with convex letters ‘LSW’, ~200 μm in thickness. LSW, Laboratory of Soft & Wet Matter. (b) Images show colour changes induced by the convex letters superimposed with a gradient stress field. The dots indicate the position where the gel undergoes the largest stress, and the brightness of the dots indicates the magnitude of the stress. (c) Mimic of an impressionist painting using photonic hydrogel, which clearly shows a boat sailing in the sea under a sunset. Different stress gradients make effects to show the boat being taken away by the incoming tide. Scale bar, 10 mm. Figure 6: A demonstration of the fast response photonic hydrogel as pressure-actuated full-colour displays. ( a ) A schematic illustration of pressure-actuated display. The elastic PDGI/h-PAAm gel ( t hydrolysis =5 min) was ~1.23 mm in thickness, and the pressure was given by a glass plate with convex letters ‘LSW’, ~200 μm in thickness. LSW, Laboratory of Soft & Wet Matter. ( b ) Images show colour changes induced by the convex letters superimposed with a gradient stress field. The dots indicate the position where the gel undergoes the largest stress, and the brightness of the dots indicates the magnitude of the stress. ( c ) Mimic of an impressionist painting using photonic hydrogel, which clearly shows a boat sailing in the sea under a sunset. Different stress gradients make effects to show the boat being taken away by the incoming tide. Scale bar, 10 mm. Full size image We report a strategy to design photonic materials with ultrafast-response and broad colour range using chemically crosslinked hydrogels imbedded with reflective platelets. Based on this strategy, we successfully developed a photonic hydrogel with thousands of rigid lamellar bilayer domains uniaxially aligned in a quasi-elastic h-PAAm hydrogel matrix. This nanostructured hydrogel exhibits mechano-actuated ultrafast colour switching over the whole visible wavelength. The rigid bilayer domains not only reflect light but also reinforce the soft gel network to give a mechanically stable material, which can sustain high-speed vibration produced by ballistic impacts and tens of thousands of high-frequency fatigue tests. These results show that the presented strategy is feasible, and can be applied to develop other novel photonic hydrogels with excellent performance. The results will expand the scope of hydrogel application in new fields, like displays and stress sensors. The small stress detecting ability in the order of kilo Pascals has potential biological applications, such as sensing the contractile force of cells by using the photonic gel as a soft scaffold. Hydrogel synthesis and hydrolysis The parent PDGI/PAAm gel with macroscopic uni-domain lamellar bilayer structure was synthesized by simultaneous free radical polymerization from aqueous solution of 0.10 M DGI, 0.027 mol% sodium dodecyl sulphate in relative to DGI, 2 M AAm, 2.5 mM N,N′-methylenebis acrylamide as a cross-linker of AAm and 2 mM Irgacure as an initiator [11] . Briefly, prior to the polymerization, by applying shear flow to the precursor solution during the injection of the solution into a reaction cell of 0.5-mm spacing, thousands of lamellar bilayers of self-assembled DGI were aligned in the direction parallel to the cell wall. To stabilize these oriented lamellar bilayers, polymerization was performed by irradiating ultraviolet light for 8 h at 50 °C under an argon gas atmosphere. After the polymerization, the gel was immersed in a large amount of water for 1 week to reach an equilibrium swelling state. The PDGI/PAAm gel have multi-bilayer structure (PDGI) stacked periodically in the PAAm matrix. The thickness of the swollen PDGI/PAAm gel was 0.97 mm. The PAAm network of the gel was hydrolyzed by treatment with 1 M sodium hydroxide aqueous solution for various times (1–6 min) at 50 °C. Before hydrolysis, the gel was immersed in 1 M sodium hydroxide at room temperature for 15 min. By the hydrolysis, the amide groups in PAAm layer (−CONH 2 ) were partially converted into carboxylate group (−COONa) ( Supplementary Fig. 5 ). The obtained hydrogel (PDGI/h-PAAm), which contains partially hydrolyzed PAAm (PAAcNa), was then extensively washed with lots of deionised water and immersed in water for >1 week to reach an equilibrium swelling state. Reflection spectrum measurement A Xe lamp was used as a light source for acquisition of the reflection spectrum. Variable angle reflection measurement optics (Hamamatsu Photonics KK, C10027A10687) were used for irradiating the gel with white light and resolving the reflected light. A photonic multichannel analyzer (Hamamatsu Photonics KK, C10027) was used for analyzing the detected signal. The entire reflection spectrum was obtained by keeping both the incident (Bragg’s angle) and reflection angles at 60°, and the maximum wavelength, λ max , was obtained from the reflection spectrum. Cyclic compressive stress−strain test The gel samples were analyzed with a commercial machine (Tensilon RTC-1310A, Orientec Co.). Samples were cut into disk-shape of 10 mm in diameter. Hysteresis was observed by performing the compressive loading followed by unloading in which the sample was initially compressed to a predefined strain and immediately unloaded to zero strain at a fixed compression increase/decrease velocity (0.5 mm s −1 ). The consecutive second hysteresis loop was performed with no waiting time after the first cycle with identical experimental conditions. Water content measurement The water content of the gel was measured using a moisture balance MOC-120H (Shimadzu Co.). The dry sample was obtained by heating the sample to 120 °C. The water content of swollen PDGI/h-PAAm hydrogel (hydrolysis time: 5 min) at 25 °C was 95%. Ballistic impacts and high-frequency fatigue test The impact strength was modulated by controlling the distance between the gel and rubber in the ballistic impact test. The whole deformation of the gel as well as the colour change was captured by a high-speed camera at 10,000 fps. The frame rate of the footage, 10,000 fps, allowed for the analysis of 125 separate images over a 12.5-ms impact release. The high-frequency fatigue test was applied under a designed oscillation system, which was subjected to some electrical circuit (150 mv) as an outside power source. The gel was periodically pressed and released at a frequency of 100 Hz. The behaviour of the gel was recorded by a high-speed camera. The colour quality of the gels in the movies taken by high-speed camera ( Supplementary Movies 3, 5 and 6 ) is not as good as the ones that were taken by a common camera ( Supplementary Movies 1, 2, 4 and 7 ). How to cite this article: Yue, Y. et al . Mechano-actuated ultrafast full-colour switching in layered photonic hydrogels. Nat. Commun. 5:4659 doi: 10.1038/ncomms5659 (2014).